Reliable reporting of Faradaic efficiencies for electrocatalysis research Thermodynamics provides a foundation for identifying potentially competing reactions in electrochemical cells. Standard reduction potentials, either measured or calculated from thermochemical data, allow a researcher to predict which reactions may occur at substantial rates at a given electrochemical potential. 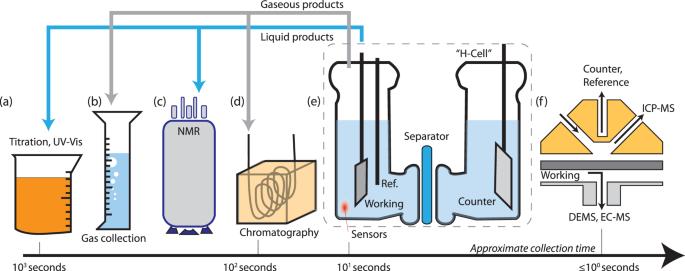Fig. 1: Instruments and methods for measuring Faradaic efficiency. Batch methods for characterizing gaseous and liquid products include titration (a), gas collection (b), NMR (c), and headspace characterization via gas chromatography (d). H-cells are used to separate the working and counter electrode for the collection of products (e). Electrochemical flow cells (f) enable nearly real-time detection of reaction and corrosion products via mass-spectrometry techniques (ICP-MS, DEMS, EC-MS). Table 1 presents the standard reduction potentials for a subset of reactions of interest to the electrocatalysis community. The measured current may be directly related to reaction rates without further analysis only when catalyst materials are thermodynamically stable and the cell is free of competing reactions and reactants (as defined by the potential of the working electrode). Notably, the ORR can interfere with nearly all other reduction reactions, requiring careful removal of O 2 from both the reaction headspace and the electrolyte. Because proton sources are required for the reactions in Table 1 , the HER may contribute substantially to the current whenever the potential is negative of the equilibrium hydrogen potential, as defined by local pH; FE measurements are essential in evaluating electrocatalysts for the CO 2 RR and N 2 RR. Table 1 Standard potentials versus the normal hydrogen electrode (NHE), reactions, and commonly employed FE measurement techniques for the proton-coupled reactions discussed in this Comment [6] , [15] , [16] Full size table Metal corrosion poses long-term stability concerns and can lead to the spontaneous generation of H 2 and other reduced products, which may lead to measured FEs greater than unity. The onset potentials for corrosion can also be predicted on thermodynamic grounds: for example, the corrosion potential of Co/Co 2+ ( E o = –0.3 V vs. the normal hydrogen electrode (NHE)) implies that Co-based electrocatalysts are likely to be passive while facilitating the HER in O 2 -free 1.0 M OH – ( E o = –0.8 V vs. NHE) but quantification of corrosion products is advisable if facilitating the HER in 1.0 M H + ( E o = 0.0 V vs. NHE). We provide the following guidance on when FE measurements should be required for publication, based on thermodynamic arguments: Could multiple products be formed at the applied potential at the working electrode? Are reactants/contaminants present in the cell environment (e.g., O 2 ) that are competitive as defined by the applied potential at the working electrode (Table 1 )? Are all components of the electrocatalyst and its support (carbon is of particular concern for OER) stable at the applied potentials and in the presence of other possible reactants and products (e.g., O 2 , H 2 O 2 , or H + )? If multiple products, including possible corrosion products, are expected, additional chemical product characterization is a critical component of catalyst activity assessment. Titrations (Fig. 1a ) are a routine method for quantifying the liquid products of bulk electrolysis. Recently, colorimetric methods (e.g., indophenol, Nessler) have seen renewed popularity in measurements of NH 3 production during the N 2 RR and other electrocatalytic NH 3 -producing processes [2] . In addition to direct analysis of the working electrolyte, researchers should first validate the sensitivity and extinction coefficient of the indicator in the presence of interferents. As a matter of practice, these colorimetric methods are not considered appropriate for monitoring trace products or when common laboratory contaminants can act as an interfering source [2] . Fig. 1: Instruments and methods for measuring Faradaic efficiency. Batch methods for characterizing gaseous and liquid products include titration ( a ), gas collection ( b ), NMR ( c ), and headspace characterization via gas chromatography ( d ). H-cells are used to separate the working and counter electrode for the collection of products ( e ). Electrochemical flow cells ( f ) enable nearly real-time detection of reaction and corrosion products via mass-spectrometry techniques (ICP-MS, DEMS, EC-MS). Full size image For gaseous products (HER, OER), selectivity has been monitored by measuring the volume of gas collected from the working electrode in an inverted burette or graduated cylinder (Fig. 1b ) [3] . One potential pitfall in this method is that it implicitly assumes that products are entirely converted to the gas phase, whereas supersaturation of the electrolyte may lead to a lower-than-expected FE. Testing at current densities >10 mA cm −2 to drive gas nucleation at the electrode surface [4] , for a sufficient duration such that headspace products greatly exceed dissolved gases, and minimizing the volume of electrolyte that can collect supersaturated gases, will lead to more accurate FE measurements. Properly calibrated electrochemical sensors (HER, OER, CO 2 RR) and fluorescence detectors (OER) in a well-stirred cell have been used to monitor the conversion of a reaction in near-real time, expressed as a rising product concentration in the electrolyte or headspace [5] . Gas chromatography (GC) and liquid chromatography (LC) are preferred for resolving dilute products produced at research-scale electrodes (Fig. 1d ). When coupled with MS, GC-MS and LC-MS allow researchers to validate that products have been derived from isotopically enriched reactants (e.g., 13 CO 2 and 15 N 2 ) [6] , [7] . Isotopically enriched products have also been resolved using NMR (Fig. 1c ) [7] to discriminate between contaminant and electrocatalytically produced N 2 RR products. Researchers must validate their ability to accurately sample the phases containing electrochemical products; errors introduced via sampling are nearly always greater than the standard error of the instrument. The inclusion of error bars, representing the standard deviation of at least three separate FE measurements, provides a more direct assessment of the measurement reproducibility. Loss of products via crossover between the working and counter electrode will lead to lower measured Faradaic efficiencies. This effect can be mitigated, but not prevented, by separating electrodes with a semipermeable membrane. For flow-through measurements, improper estimation of gas flow is commonly observed for the dissolution of CO 2 into aqueous, alkaline electrolytes, which leads to greater-than-expected concentrations of products and overestimations of the FE [8] . Precise downstream measurements of volume flow, near the instrument sampling product concentrations, are recommended. When the sum of all product FEs is significantly less than 100%, researchers may investigate escaped products, consumption at the counter electrode, and homogeneous reactions within the cell; total FEs greater than 100% may be due to overestimation of sampled volume, sampling a preconcentrated product, or spontaneous generation of product through a chemical reaction (e.g., corrosion). Direct collection of electrolyte volumes near the electrode surface can enable a continuous analysis of products such that the measured FE approximates the current efficiency (CE). We endorse a textbook distinction of CE, which refers to the instantaneous selectivity toward a specific half-reaction [1] , although FE and CE have often been used interchangeably. For kinetically facile 2e – reactions, rotating-ring disc electrodes (RRDE) combine a generator electrode (the disc) with a collector electrode (the ring) to simultaneously measure reaction rates and product selectivity at equivalent time scales. This method has been classically used for quantifying the FE between the 2e – and 4e – pathways of the ORR [9] (Table 1 ) and, more recently, was used to monitor the FE and local pH shift during CO 2 RR at an Au surface [10] . The collection efficiency of the ring should be carefully calibrated using a one-electron redox couple (e.g., Fe(CN) 6 4 – /Fe(CN) 6 3 – ) in the supporting electrolyte of interest. MS tools coupled to electrochemical flow cells (e.g., differential electrochemical MS [DEMS] or electrochemical MS [EC-MS], Fig. 1f ) improve temporal resolution in FE measurements by detecting changes in the mass-selected signal of products collected adjacent to the working electrode surface. Because the relationship between ion current and FE is itself ambiguous, careful reporting of the calibration method (either via standard samples or a cell environment with FE ~ 1) is important. This method has been used to simultaneously measure hydrogen, hydrocarbons, and oxygenates produced at a Cu thin film [11] , [12] and has also been used to monitor corrosion reactions at carbon supports [13] . For aqueous corrosion products, online inductively coupled plasma MS (ICP-MS, Fig. 1f ) has correlated corrosion data within seconds of changes in the applied potential [14] . Such measurements are critical for assessing the commercial viability of catalysts free of (or with low loadings of) platinum group metals and researchers measuring Faradaic efficiencies should not restrict their focus toward measurements of product selectivity but rather all of the electrochemical reactions occurring at the interface of interest. Transparency in electrocatalysis research is critical and is supported by detailed descriptions of the methods used to measure FE. Reporting reactor volumes and sampled volumes for batch measurements and flow rates leaving a reactor for online measurements are good practices to allow readers and reviewers to independently assess the measurement. Control experiments using electrocatalysts with established activity and selectivity and/or labeled reactants are effective for measuring reproducibility and sources of systematic error. In summary, the burden of proof is on the researcher to connect ambiguous electrochemical data to the assumed chemical reaction of interest. Inexpensive approaches involving titrations and gas collection are sufficiently accessible that some form of FE measurement should be connected to any electrochemical current that may be assigned to more than one half-reaction. Through hydrodynamic control of the electrolyte at the electrocatalyst surface, modern FE measurements now approach real-time quantification of products, facilitating more-robust reporting of catalyst activity, selectivity and stability.